VEGETATIVE1is essential for development of the compound inflorescence in pea Unravelling the basis of variation in inflorescence architecture is important to understanding how the huge diversity in plant form has been generated. Inflorescences are divided between simple, as in Arabidopsis, with flowers directly formed at the main primary inflorescence axis, and compound, as in legumes, where they are formed at secondary or even higher order axes. The formation of secondary inflorescences predicts a novel genetic function in the development of the compound inflorescences. Here we show that in pea this function is controlled by VEGETATIVE1 ( VEG1 ), whose mutation replaces secondary inflorescences by vegetative branches. We identify VEG1 as an AGL79 -like MADS-box gene that specifies secondary inflorescence meristem identity. VEG1 misexpression in meristem identity mutants causes ectopic secondary inflorescence formation, suggesting a model for compound inflorescence development based on antagonistic interactions between VEG1 and genes conferring primary inflorescence and floral identity. Our study defines a novel mechanism to generate inflorescence complexity. Understanding the basis of diversity in form is a major challenge in developmental biology. An important feature contributing to form diversity in angiosperms is the variation in the architecture of inflorescences, the structures that bear the flowers [1] , [2] . Inflorescence architecture is also important because it conditions flower and fruit production and, therefore, crop yield [3] . A process central to generation of inflorescence architecture diversity is inflorescence branching, with a major distinction between simple inflorescences, as in Arabidopsis, where flowers derive from the primary inflorescence axis ( Fig. 1a,b,c), and compound inflorescences, where flowers form at secondary (or higher order) branches ( Fig. 1d,e,f ) [2] . 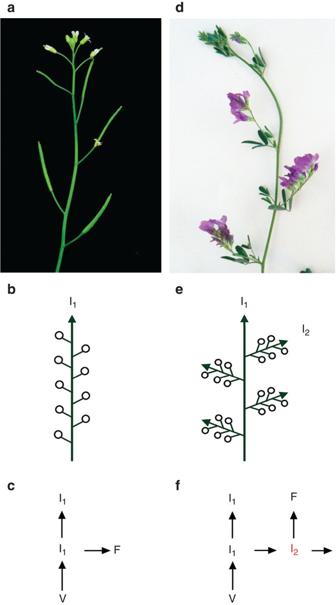Figure 1: Examples of simple and compound inflorescences. (a) Simple raceme ofArabidopsis thaliana. (b) Diagram of the architecture of the inflorescence showed in (a). (c) Schematic representation of meristem identity in the inflorescence showed in (a). (d) Compound raceme of the legume speciesMedicago sativa. (e) Diagram of the architecture of the inflorescence showed in (d). (f) Schematic representation of meristem identity in the inflorescence showed in (d). In Arabidopsis, flowers appear in the primary inflorescence stem (I1) whereas inM. sativathey appear in secondary inflorescence branches (I2). V, vegetative meristem; I1, primary inflorescence meristem; I2, secondary inflorescence meristem; F, floral meristem. Figure 1: Examples of simple and compound inflorescences. ( a ) Simple raceme of Arabidopsis thaliana . ( b ) Diagram of the architecture of the inflorescence showed in ( a ). ( c ) Schematic representation of meristem identity in the inflorescence showed in ( a ). ( d ) Compound raceme of the legume species Medicago sativa . ( e ) Diagram of the architecture of the inflorescence showed in ( d ). ( f ) Schematic representation of meristem identity in the inflorescence showed in ( d ). In Arabidopsis, flowers appear in the primary inflorescence stem (I 1 ) whereas in M. sativa they appear in secondary inflorescence branches (I 2 ). V, vegetative meristem; I 1 , primary inflorescence meristem; I 2 , secondary inflorescence meristem; F, floral meristem. Full size image Genetic control of compound inflorescence development has been best studied in grasses, particularly in rice and maize, where flowers are formed from the spikelet meristem, an inflorescence meristem that frequently derives from lateral secondary or tertiary order inflorescence branches [4] , [5] . This higher complexity suggests that novel genetic functions must exist for the formation of the high-order inflorescence meristems, that often are not simple reiterations of the primary inflorescence meristem. In fact, a number of genes have been characterized that control specific aspects of compound inflorescence development in grasses, such as the formation of lateral inflorescences or the determinacy of spikelet meristems [4] , [5] , [6] , [7] . Compound inflorescence development has also been studied in Solanaceae, where two genes that control inflorescence complexity have been isolated. However, the formation of Solanaceae compound inflorescences differs from grasses, not involving high-order inflorescence meristems [8] . Legumes (Fabaceae), the third largest angiosperm family, also have compound inflorescences [9] , [10] , where flowers are produced on lateral secondary inflorescence branches ( Fig. 1d,e,f ). In this respect, legume inflorescence architecture is similar to that of grasses and different to Solanaceae. Given that legumes are only distantly related to grasses, a relevant question is whether legumes have generated secondary inflorescence meristems through a distinct mechanism involving novel specific functions. To understand the development of the compound inflorescence in legumes, we analysed the classical vegetative1 ( veg1 ) mutant from pea ( Pisum sativum ), which displays a phenotype that suggests severe defects in the formation of secondary inflorescence meristems [11] , [12] , and, therefore, we hypothesized that it might be defective in such novel function. VEG1 is required to make secondary inflorescences The pea inflorescence is a compound raceme, typical of many legumes [1] , [10] , [13] . During the vegetative phase, each of the nodes produced by the vegetative shoot apical meristem (SAM) consists of a leaf with a shoot axillary meristem that generally remains dormant until the floral transition has occurred ( Fig. 2a–c ). At floral transition, the SAM becomes a primary inflorescence (I 1 ) meristem, with indeterminate growth, that produces nodes with axillary meristems that grow out immediately ( Fig. 2a–c ). These secondary inflorescence (I 2 ) meristems each produce 1–3 nodes bearing floral meristems before terminating in a stub [1] , [13] ( Fig. 2d ). Therefore, the I 2 meristem, interposed between the I 1 and the floral meristems, represents an additional level of complexity compared with the simple raceme of Arabidopsis ( Fig. 1c ). 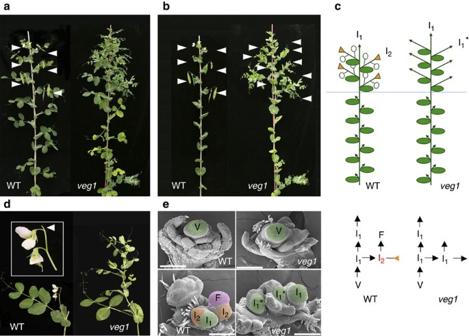Figure 2: Mutant secondary inflorescences replaced by vegetative branches in peaveg1. (a) Pea wild-type (WT) andveg1plants grown for 11 weeks. Whereas the upper nodes of the wild type contain secondary inflorescences (I2) with flowers (pods, arrowheads),veg1has not produced any flower. (b) The same plants as in (a), where leaves have been removed. As in the wild type, the axillary buds of the lower nodes ofveg1remain dormant. However, at the nodes where I2s (arrowheads) have grown in the wild type, branches (arrowheads) have grown out inveg1. (c) Diagrams (top) and schematic representation of meristem identity (bottom) of the wild-type andveg1mutant plants. The vegetative meristem (V) becomes a primary inflorescence meristem (I1) that produces secondary inflorescence meristems (I2) that form flowers (F). In theveg1plants the I2s are replaced by vegetative branches similar to I1s (I1*). Arrowheads, indeterminate shoots; open circles, flowers; orange triangles, stubs. (d) Structures formed in equivalent apical nodes of the inflorescence stems of wild-type andveg1plants. Whereas the wild type has produced an I2with two flowers and a stub (arrowhead in inset),veg1has produced a vegetative branch. (e) Scanning electron micrographs of the main shoot apex of wild type andveg1. During the vegetative phase (top), in both the wild type andveg1, the vegetative SAM (V, highlighted in green) generates leaves with dormant axillary meristems. After transition to flowering (bottom), the SAM in the wild type becomes a primary inflorescence meristem (I1) that produces I2meristems (orange) with floral meristems (F, pink). At an equivalent developmental stage, the SAM ofveg1produces leaves with axillary meristems (I1*, green) that grow out following the same pattern as the I1meristem. Scale bars, 200 μm. Figure 2: Mutant secondary inflorescences replaced by vegetative branches in pea veg1 . ( a ) Pea wild-type (WT) and veg1 plants grown for 11 weeks. Whereas the upper nodes of the wild type contain secondary inflorescences (I 2 ) with flowers (pods, arrowheads), veg1 has not produced any flower. ( b ) The same plants as in ( a ), where leaves have been removed. As in the wild type, the axillary buds of the lower nodes of veg1 remain dormant. However, at the nodes where I 2 s (arrowheads) have grown in the wild type, branches (arrowheads) have grown out in veg1 . ( c ) Diagrams (top) and schematic representation of meristem identity (bottom) of the wild-type and veg1 mutant plants. The vegetative meristem (V) becomes a primary inflorescence meristem (I 1 ) that produces secondary inflorescence meristems (I 2 ) that form flowers (F). In the veg1 plants the I 2 s are replaced by vegetative branches similar to I 1 s (I 1 *). Arrowheads, indeterminate shoots; open circles, flowers; orange triangles, stubs. ( d ) Structures formed in equivalent apical nodes of the inflorescence stems of wild-type and veg1 plants. Whereas the wild type has produced an I 2 with two flowers and a stub (arrowhead in inset), veg1 has produced a vegetative branch. ( e ) Scanning electron micrographs of the main shoot apex of wild type and veg1 . During the vegetative phase (top), in both the wild type and veg1 , the vegetative SAM (V, highlighted in green) generates leaves with dormant axillary meristems. After transition to flowering (bottom), the SAM in the wild type becomes a primary inflorescence meristem (I 1 ) that produces I 2 meristems (orange) with floral meristems (F, pink). At an equivalent developmental stage, the SAM of veg1 produces leaves with axillary meristems (I 1 *, green) that grow out following the same pattern as the I 1 meristem. Scale bars, 200 μm. Full size image The vegetative1 ( veg1 ) mutant derives from X-ray mutagenesis [11] , and, among numerous flowering-related mutants in pea, it is distinctive in that it never produces flowers under any conditions ( Fig. 2a ), and may persist in a vegetative state for over 6 months under conditions where wild-type plants flower after several weeks [12] . During the vegetative phase, veg1 and wild-type plants were indistinguishable, with dormant axillary meristems ( Fig. 2a–c,e ). However, after the floral transition, nodes equivalent to those occupied by I 2 s in wild type were also released from dormancy in veg1 , but produced only vegetative shoots ( Fig. 2a,b,d,e ; Supplementary Fig. S1 ). This suggests that veg1 mutants undergo a phase transition but are impaired in the subsequent specification of secondary inflorescence identity. To test this possibility, we compared the expression of inflorescence markers in wild type and veg1 . In wild-type plants, the floral transition is associated with transcriptional induction of DETERMINATE ( DET ) and PROLIFERATING INFLORESCENCE MERISTEM ( PIM ) [14] , [15] , [16] , [17] ( Fig. 3a ), which, like their Arabidopsis orthologues TERMINAL FLOWER 1 ( TFL1 ) [18] and APETALA 1 ( AP1 ) [19] , control the identity of the inflorescence and the floral meristems [14] , [15] , [17] , [18] , [19] , [20] . In 5-week-old plants, where PIM is clearly expressed in wild-type plants, expression was not observed in veg1 ( Fig. 3a ), consistent with the absence of flowers or floral organs. However, the inflorescence marker DET was upregulated in veg1 similarly to wild type. Taken together, these results support the idea that the apex of veg1 plants go through floral transition at approximately the same time as the wild type. This implies that the extreme non-flowering phenotype of the veg1 mutant plants does not represent a block in floral induction or a defect in timing of the floral transition, but instead reflects a failure of the lateral meristems produced by the primary 'inflorescence' apex of veg1 to develop as secondary inflorescences. Therefore, VEG1 is required for the pea inflorescence apex to make the I 2 meristems. 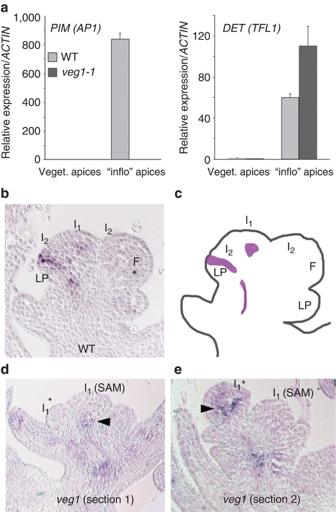Figure 3: Expression of meristem identity genes in the shoot apex ofveg1. (a) mRNA levels ofPIM(left) andDET(right) in the shoot apices of the wild type andveg1. Relative mRNA levels were determined by RT–qPCR. Samples were from main-shoot apices of 2-week old plants (veget. apices), before wild-type plants had gone through the floral transition, and of 5-week-old plants ('inflo' apices), when the wild type had started producing flowers. Values represent the means of two biological replicates ±s.e. (b–e)In situhybridization ofDETmRNA in the shoot apices of wild type andveg1. Samples were from the main apices of 4-week-old plants, when the wild type had gone through the floral transition. In the wild-type apex (b)DETexpression was detected below the dome of the primary inflorescence meristem (I1), in the vasculature, and in the boundary between the secondary inflorescence meristem (I2) and the incipient leaf primordium (LP), but not in the I2or in the floral meristems (F), as represented in the diagram (c), for clarity. Similarly, inveg1, expression was also detected below the primary shoot meristem (I1SAM, arrowhead), in a section through the centre of the apex (d). A deeper section from the same apex (e) shows that inveg1 DETis also expressed in a lateral shoot meristem (I1*, arrowhead). Figure 3: Expression of meristem identity genes in the shoot apex of veg1 . ( a ) mRNA levels of PIM (left) and DET (right) in the shoot apices of the wild type and veg1 . Relative mRNA levels were determined by RT–qPCR. Samples were from main-shoot apices of 2-week old plants (veget. apices), before wild-type plants had gone through the floral transition, and of 5-week-old plants ('inflo' apices), when the wild type had started producing flowers. Values represent the means of two biological replicates ±s.e. ( b–e ) In situ hybridization of DET mRNA in the shoot apices of wild type and veg1 . Samples were from the main apices of 4-week-old plants, when the wild type had gone through the floral transition. In the wild-type apex ( b ) DET expression was detected below the dome of the primary inflorescence meristem (I 1 ), in the vasculature, and in the boundary between the secondary inflorescence meristem (I 2 ) and the incipient leaf primordium (LP), but not in the I 2 or in the floral meristems (F), as represented in the diagram ( c ), for clarity. Similarly, in veg1 , expression was also detected below the primary shoot meristem (I 1 SAM, arrowhead), in a section through the centre of the apex ( d ). A deeper section from the same apex ( e ) shows that in veg1 DET is also expressed in a lateral shoot meristem (I 1 *, arrowhead). Full size image To elucidate the nature of the vegetative branches that replace the I 2 s in the veg1 mutant, we further analysed the expression of DET , in more detail, by in situ hybridization. In wild-type apices, DET expression was restricted to the primary inflorescence meristem ( Fig. 3b,c ). However, in veg1 apices DET was expressed not only in the I 1 meristem but also in the lateral meristems that are formed in place of the I 2 meristems ( Fig. 3d,e ). This indicates that the lateral branches produced by veg1 plants after the transition possess I 1 identity, and further supports a role for VEG1 in the specification of I 2 identity ( Fig. 2c ). Although VEG1 , thus, seems required for the specification of I 2 meristems, a further question concerns whether it is also required for the formation of flowers. In contrast to the constitutive non-flowering phenotype of the veg1 mutant, the veg1 det double mutant does produce flowers [13] ( Supplementary Fig. S2a,b ). However, in contrast to the det single mutant, where the primary inflorescence ends in a terminal I 2 , the veg1 det primary inflorescence does not produce I 2 s, and ends with the production of a terminal flower, often after producing a flower directly from the axil of a leaf at the node below [13] ( Supplementary Fig. S2c-f ). Consistent with that, we saw that expression of PIM is induced in the apex of veg1 det plants ( Supplementary Fig. S2g,h ). This again indicates that VEG1 is required for the specification of the I 2 meristems, and shows that it is not directly required for the expression of the floral meristem identity genes or the formation of floral meristems. VEG1 is a MADS-box gene from the AGL79 clade To identify a candidate gene for VEG1 , we adopted a comparative mapping strategy using the related model legume Medicago truncatula , which has inflorescence architecture identical to pea [21] . The VEG1 locus was initially observed to map to the bottom of pea linkage group V (top of Medicago chromosome 7), near the MADS-box gene PsSEPALLATA1 ( PsSEP1 ) [22] , and we found that this gene was deleted in veg1 . However, consistent with the well-documented role for SEP genes in floral organ identity [23] , [24] , we found that PsSEP1 was expressed in floral but not in I 2 meristems, thus arguing against PsSEP1 as a candidate for VEG1 . In M. truncatula , a second MADS-box gene, MtFULc , is located on the same BAC clone as MtSEP1 (ref. 22 ) ( Fig. 4a ). We isolated the pea orthologue of this gene ( PsFULc ), confirmed its map position very close to PsSEP1 , and observed that it is also deleted in the veg1 mutant ( Fig. 4b ). PsFULc and MtFULc belong to the AGL79 clade of the AP1/SQUA/FUL genes [25] , [26] ( Supplementary Fig. S3 ). Genes from the AP1/SQUA/FUL lineage are involved in the specification of meristem identity [20] , which suggested that PsFULc was a good candidate for VEG1 . 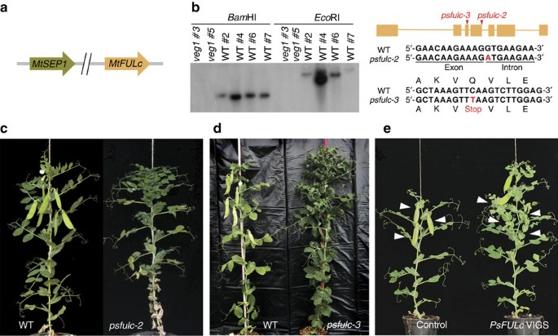Figure 4: Cloning ofVEG1. (a) InM. truncatula,MtFULcis located 17 Kb fromMtSEP1, whose pea homologue maps to theVEG1locus and is deleted in theveg1mutant. (b) Lesions in thepsfulcmutant alleles described in this work. Left, Southern blot on DNA of plants from a F2 population segregating forveg1, hybridized with aPsFULcprobe. The same DNA samples were digested withBamHI and withEcoRI. Hybridization was observed with DNA from plants with a wild-type phenotype (2, 4, 6 and 7) but not from homozygousveg1plants (3 and 5), showing thatPsFULcis deleted inveg1. Right, mutations in thepsfulc-2andpsfulc-3alleles. The nucleotide changes in the mutant sequences are indicated in red. The G-to-A mutation infulc-2destroyed the splice donor site of exon 3. The C-to-T mutation inpsfulc-3caused a Q102STOP change. (c,d) Phenotype of thepsfulc-2andpsfulc-3mutant plants. Both plants show a non-floweringveg1phenotype, where secondary inflorescences (I2) are replaced by vegetative branches. (e)veg1-like phenotype of aPsFULc-VIGS plant. In thePsFULc-silenced plant, the I2s appear in later nodes than in the control plant, and branches (arrowheads) develop in the nodes where I2s (arrowheads) appear in the control plant. Figure 4: Cloning of VEG1 . ( a ) In M. truncatula , MtFULc is located 17 Kb from MtSEP1 , whose pea homologue maps to the VEG1 locus and is deleted in the veg1 mutant. ( b ) Lesions in the psfulc mutant alleles described in this work. Left, Southern blot on DNA of plants from a F2 population segregating for veg1 , hybridized with a PsFULc probe. The same DNA samples were digested with Bam HI and with Eco RI. Hybridization was observed with DNA from plants with a wild-type phenotype (2, 4, 6 and 7) but not from homozygous veg1 plants (3 and 5), showing that PsFULc is deleted in veg1 . Right, mutations in the psfulc-2 and psfulc-3 alleles. The nucleotide changes in the mutant sequences are indicated in red. The G-to-A mutation in fulc-2 destroyed the splice donor site of exon 3. The C-to-T mutation in psfulc-3 caused a Q102STOP change. ( c , d ) Phenotype of the psfulc-2 and psfulc-3 mutant plants. Both plants show a non-flowering veg1 phenotype, where secondary inflorescences (I 2 ) are replaced by vegetative branches. ( e ) veg1 -like phenotype of a PsFULc -VIGS plant. In the PsFULc -silenced plant, the I 2 s appear in later nodes than in the control plant, and branches (arrowheads) develop in the nodes where I 2 s (arrowheads) appear in the control plant. Full size image To assess whether the deletion of PsFULc was the cause of the veg1 phenotype, we characterized additional mutant alleles of PsFULc . Forward screening of an ethyl methanesulfonate (EMS)-mutagenized population [27] identified a single M 2 plant in which secondary inflorescences were replaced by vegetative branches, as in veg1 ( Fig. 4c ). Sequencing of PsSEP1 - and PsFULc -coding regions in this mutant ( psfulc-2 ) revealed a wild-type PsSEP1 sequence, but identified a G-to-A mutation typical of EMS mutagenesis at the 5′-splice junction of the fourth intron in PsFULc ( Fig. 4b ). A third PsFULc mutant allele ( psfulc-3 ), carrying a Q102STOP mutation, was identified in reverse genetic screening of an EMS-mutagenized Targeting-Induced Local Lesions in Genomes (TILLING) population [28] . Like psfulc-2 , this mutant also showed a clear veg1 phenotype ( Fig. 4d ) and carried a PsSEP1 -coding region identical to wild type. As a third line of evidence, we used virus-induced gene silencing (VIGS) [29] to specifically suppress expression of PsFULc , and found that PsFULc -VIGS plants partly phenocopied the veg1 phenotype. The node at which the first I 2 appeared was significantly higher in PsFULc -VIGS plants (14.5±1.6) than in control plants (10.7±0.9) and the intervening nodes were occupied by vegetative branches ( Fig. 4e ; Supplementary Fig. S1 ), as in veg1 plants. In summary, the phenotype of the PsFUL c-VIGS plants, and the defects of psfulc-2 and psfulc-3 , identical to those of the original veg1 X-ray mutant, show that the veg1 phenotype is specifically caused by the loss of PsFULc and that the deletion of other sequences in the X-ray veg1 mutant does not significantly contribute to it. Therefore, we subsequently refer to PsFULc as VEG1 . VEG1 expression marks secondary inflorescence meristems To assess whether the expression of VEG1 is consistent with its proposed role in the specification of I 2 meristem identity, we examined its expression pattern in wild-type plants and in mutants either completely lacking or producing ectopic secondary inflorescences. Analysis by RT–qPCR in wild-type plants showed that VEG1 is expressed in inflorescence apices and mature flowers ( Supplementary Fig. S4a ). Consistent with that, a time-course expression analysis showed that VEG1 upregulation occurs during the floral transition, after FTb2 , a leaf marker of floral induction [16] , and before the floral meristem identity gene PIM ( Supplementary Fig. S4b ). Further analysis by in situ hybridization on wild-type inflorescence apices ( Fig. 5a,b ) showed that VEG1 is expressed in the I 2 meristems but is not expressed in the apical meristem of the primary inflorescence (I 1 ) or in the young floral meristems, which show strong expression of PIM ( Fig. 5c,d ). These results further support the idea that VEG1 specifies the identity of I 2 meristems. 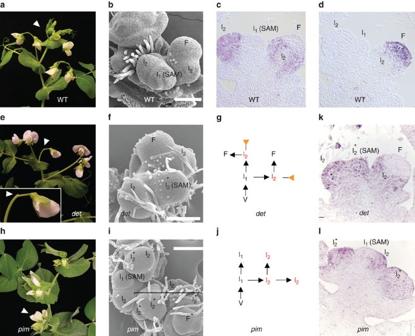Figure 5:VEG1is expressed in I2meristems of wild type and in ectopic I2meristems of pea inflorescence mutants. (a) Inflorescence of a pea wild-type plant. The inflorescence apex (arrowhead) exhibits indeterminate growth. (b) SEM image showing the different meristem types in a wild-type inflorescence. The SAM is a primary inflorescence (I1) meristem that has produced secondary inflorescence (I2) meristems, one of which has produced a floral meristem (F). (c)In situhybridization ofVEG1mRNA in the inflorescence apex of the wild type.VEG1is expressed in the lateral I2meristems, not in the I1neither in the floral meristem (F). (d)In situhybridization ofPIMmRNA in the wild-type inflorescence, in a contiguous section to that in (c). ThePIMsignal is observed only in the floral meristem, which does not expressVEG1. (e) Inflorescence of adetmutant, where the apex has converted into an I2(arrowhead). The terminal I2stem subtends a flower and ends into a stub (arrowhead in inset). (f) SEM image of adetinflorescence apex. The SAM has the characteristic shape of an I2meristem (I2*). (g) Schematic representation of meristem identity in thedetinflorescence. V, vegetative meristem; orange triangles, stubs. (h) Inflorescence of apimmutant, showing proliferative I2s (arrowhead) with abnormal flowers. (i) SEM image of apiminflorescence apex, showing I2s that, rather than flowers, produce new I2s (I2*). One of the proliferative I2s is producing a floral primordium (F*). (j) Schematic representation of meristem identity in thepiminflorescence. (k)In situhybridization ofVEG1mRNA in the inflorescence apex ofdet. In thedetmutantVEG1is also expressed in the SAM (I2*), which is converted into an I2. (l)In situhybridization ofVEG1mRNA in the inflorescence apex ofpim. Expression ofVEG1is observed not only in the lateral I2s but also in the meristem being formed by the I2at the right (I2*), which is converted from a floral meristem to an I2meristem. Scale bars, 100 μm. Figure 5: VEG1 is expressed in I 2 meristems of wild type and in ectopic I 2 meristems of pea inflorescence mutants. ( a ) Inflorescence of a pea wild-type plant. The inflorescence apex (arrowhead) exhibits indeterminate growth. ( b ) SEM image showing the different meristem types in a wild-type inflorescence. The SAM is a primary inflorescence (I 1 ) meristem that has produced secondary inflorescence (I 2 ) meristems, one of which has produced a floral meristem (F). ( c ) In situ hybridization of VEG1 mRNA in the inflorescence apex of the wild type. VEG1 is expressed in the lateral I 2 meristems, not in the I 1 neither in the floral meristem (F). ( d ) In situ hybridization of PIM mRNA in the wild-type inflorescence, in a contiguous section to that in ( c ). The PIM signal is observed only in the floral meristem, which does not express VEG1 . ( e ) Inflorescence of a det mutant, where the apex has converted into an I 2 (arrowhead). The terminal I 2 stem subtends a flower and ends into a stub (arrowhead in inset). ( f ) SEM image of a det inflorescence apex. The SAM has the characteristic shape of an I 2 meristem (I 2 *). ( g ) Schematic representation of meristem identity in the det inflorescence. V, vegetative meristem; orange triangles, stubs. ( h ) Inflorescence of a pim mutant, showing proliferative I 2 s (arrowhead) with abnormal flowers. ( i ) SEM image of a pim inflorescence apex, showing I 2 s that, rather than flowers, produce new I 2 s (I 2 *). One of the proliferative I 2 s is producing a floral primordium (F*). ( j ) Schematic representation of meristem identity in the pim inflorescence. ( k ) In situ hybridization of VEG1 mRNA in the inflorescence apex of det . In the det mutant VEG1 is also expressed in the SAM (I 2 *), which is converted into an I 2 . ( l ) In situ hybridization of VEG1 mRNA in the inflorescence apex of pim . Expression of VEG1 is observed not only in the lateral I 2 s but also in the meristem being formed by the I 2 at the right (I 2 *), which is converted from a floral meristem to an I 2 meristem. Scale bars, 100 μm. Full size image Mutations in DET or PIM , homologues of TFL1 and AP1 , respectively, cause the conversion of other meristems of the pea inflorescence into I 2 meristems. Thus, while the primary inflorescence meristem (the inflorescence SAM) of wild-type pea plants shows indeterminate growth, producing I 2 s only in lateral positions ( Figs 2c and 5a ), in det mutants, the inflorescence SAM shows determinate growth, and terminates in a typical I 2 (refs. 15 , 30 ) ( Fig. 5e,f,g ). On the other hand, the lateral meristems in the I 2 of pim mutant plants, rather than acquiring floral identity, as in the wild type ( Figs 2c and 5b ), retain I 2 meristem identity and themselves generate lateral meristems with I 2 identity in a reiterative manner, with some of these supernumerary I 2 meristems eventually producing flowers [17] , [30] ( Fig. 5h,i,j ). If VEG1 specifies I 2 identity, it would be expected that the formation of the ectopic I 2 meristems in these mutants were accompanied by changes in VEG1 expression. In fact, in situ hybridization showed that in the det mutant inflorescence VEG1 is expressed not only in the lateral I 2 meristems but also in the apical meristem ( Fig. 5k ), and that the supernumerary I 2 meristems in the pim mutant exhibit VEG1 expression ( Fig. 5l ). This indicates that DET and PIM repress VEG1 expression and restrict it to the I 2 , and suggests that the ectopic expression of VEG1 in det and pim mutants causes the conversion of I 1 and floral meristems, respectively, into I 2 meristems. Severe mutations in the VEGETATIVE2 ( VEG2 ) or GIGAS genes cause a non-flowering phenotype similar to the veg1 mutant ( gigas only under long-day photoperiods), with no formation of secondary inflorescences [16] , [31] . As in veg1 , the plants of both mutants show outgrowth of vegetative lateral branches at nodes occupied in wild-type plants by I 2 s (ref. 16 ) (Sussmilch et al ., unpublished). This similarity suggests that these genes participate in the same genetic network as VEG1 and raises the question of what is their relative position in that network. Analysis by RT–qPCR showed that although VEG1 was upregulated in shoot apices of 4-week-old wild-type plants, its expression was not detectable in either mutant ( Supplementary Fig. S4c ) after 6 weeks. This indicates that VEG1 acts downstream of VEG2 and GIGAS and suggests that they participate in the activation of VEG1 expression. This seems particularly likely for GIGAS [16] , in view of the fact that its Arabidopsis homologue FLOWERING LOCUS T ( FT) is a direct activator of the floral identity genes AP1 and FUL [32] , [33] , [34] , [35] , which are MADS-box genes from the same lineage as VEG1 ( Supplementary Fig. S3 ). Our data suggest a genetic model that explains the specification of the identity of the different meristem types formed in the pea compound inflorescence ( Fig. 6a ). In this model, expression of VEG1 , which is required to specify I 2 identity, is restricted to the I 2 meristem by DET , which represses it in the I 1 meristem, and by PIM , which represses it in the floral meristem. Conversely, expression of DET itself is restricted to the I 1 and excluded from the I 2 through repression by VEG1 . The simplest interpretation of the veg1 phenotype is, therefore, that it results from ectopic DET expression in the lateral I 2 meristems, converting them into I 1 meristems ( Fig. 6b ). In addition, the formation of flowers in the veg1 det double mutant suggests that DET represses not only VEG1 but also PIM expression. Finally, the fact that the flowers in veg1 det are directly formed from the I 1 , as in simple inflorescences, suggests that the default state of the meristems in the pea inflorescence is floral identity, which is normally restricted to the lateral meristems of the I 2 by the concerted action of DET and VEG1. In this sense, VEG1 would be required to maintain 'vegetativeness', as defined by Prusinkiewicz et al . [36] , in the lateral meristems of the I 1 . 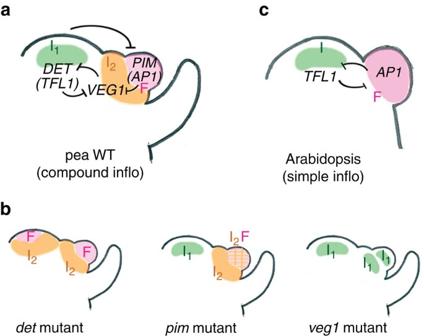Figure 6: Genetic model for specification of meristem identity in the compound inflorescence of pea. (a) In the pea compound inflorescence, expression ofDET(orthologue ofTFL1) in the I1,VEG1in the I2andPIM(orthologue ofAP1) in the floral meristems are required for those meristems to acquire their identity. Expression of these genes in their correct domains is maintained by a network of mutual repressive interactions. (b) The genetic model explains the phenotypes of the pea meristem identity mutants. The absence ofDETin thedetmutant allows expression ofVEG1in the SAM, which gets converted into an I2. The absence ofPIMallows the expression ofVEG1in the floral meristem, which gets converted into a proliferative I2. In absence ofVEG1,DETis expressed in all the meristems in the apex, and they get converted into I1s. (c) Meristem identity in the simple inflorescence of Arabidopsis is maintained by a similar genetic network than in pea, butVEG1function is absent and I2meristem is not formed. Figure 6: Genetic model for specification of meristem identity in the compound inflorescence of pea. ( a ) In the pea compound inflorescence, expression of DET (orthologue of TFL1 ) in the I 1 , VEG1 in the I 2 and PIM (orthologue of AP1 ) in the floral meristems are required for those meristems to acquire their identity. Expression of these genes in their correct domains is maintained by a network of mutual repressive interactions. ( b ) The genetic model explains the phenotypes of the pea meristem identity mutants. The absence of DET in the det mutant allows expression of VEG1 in the SAM, which gets converted into an I 2 . The absence of PIM allows the expression of VEG1 in the floral meristem, which gets converted into a proliferative I 2 . In absence of VEG1 , DET is expressed in all the meristems in the apex, and they get converted into I 1 s. ( c ) Meristem identity in the simple inflorescence of Arabidopsis is maintained by a similar genetic network than in pea, but VEG1 function is absent and I 2 meristem is not formed. Full size image The network of mutually repressive interactions between DET , VEG1 and PIM resembles the simpler genetic network that controls meristem identity in the inflorescence apex of Arabidopsis ( Fig. 6c ), where the separation of the inflorescence and floral meristematic domains is achieved by mutual repression between TFL1 and the floral meristem genes AP1 and LEAFY ( LFY ) [20] . This similarity suggests a mechanism in which evolutionary modification of a simple raceme (for example, Arabidopsis) into a compound form may have occurred through the appearance of a new function, VEG1 , acting between the inflorescence identity function of DET ( TFL1 ) and the floral identity function of PIM ( AP1 ), which leads to the formation of a new intermediate-step meristem, the I 2 , and therefore to the development of a compound inflorescence. The VEG1 gene belongs to the AP1/SQUA/FUL lineage, represented in core eudicots by three distinct clades, eu AP1 , eu FUL and AGL79 , that likely arose from a common eudicot ancestor through duplication [25] , [26] . While no functional information from mutant phenotypes is available for any AGL79 -like gene, analysis of several euAP1 genes and of the Arabidopsis eu FUL gene FRUITFULL ( FUL ) indicates that genes in these other sub-clades control the identity of reproductive meristems [20] , [37] . This suggests that this basic function was already present in the ancestor of the core-eudicot AP1/SQUA/FUL genes, and we speculate that AGL79 genes, such as VEG1 , may have sub-functionalized to specify the identity of I 2 meristems. Is the mechanism of I 2 identity specification, through VEG1 -like genes, also central for compound inflorescence development in species other than pea? Compound inflorescences are widespread in the Fabaceae family, suggesting a common evolutionary origin. As VEG1 orthologues are found in several papillionoid legumes ( Supplementary Fig. S3 ), and more widely in eudicots, it seems likely that VEG1 function was present early in the evolution of Fabaceae and may have arisen before the origin of this group. However, no monocot orthologue exists for VEG1/AGL79 , a core-eudicot-specific gene [25] , [26] , and consistent with this, the genetic network controlling compound inflorescence formation in grasses is different to that in legumes and does not seem to involve a VEG1 -related function [4] , [5] , [6] , [7] , [38] . Within the eudicots, compound inflorescences have also been studied in Solanaceae [8] , but, in this group, the ontogeny of the compound inflorescence does not involve high-order inflorescence meristems [8] and is thus quite distinct from that in either legumes or grasses. Accordingly, the genes known to control complexity in this family are distinct from those in legumes and grasses and also do not include a VEG1 orthologue [8] . Thus, these groups apparently use distinct genetic networks for inflorescence complexity, suggesting that compound inflorescences have independently appeared several times during angiosperm evolution. This is consistent with the fact that compound inflorescences occur in phylogenetically distant plant families [2] . In summary, our work provides the first insight into the genetic network controlling the legume compound inflorescence. We identify a novel mechanism for generation of inflorescence complexity, distinct from that in grasses and Solanaceae, which is based on the function of the VEG1 gene, which acts between the I 1 and floral meristem identity genes to specify formation of the I 2 meristem. The identification of VEG1 as an AGL79 -like MADS-box gene suggests that VEG1 function derives from sub-functionalization of the AGL79 clade within the eudicot AP1/SQUA/FUL genes. More generally, our identification of VEG1 provides an illustration of how the expansion and functional divergence within key regulatory gene families can contribute to the evolution of morphological complexity. Plant material and growth conditions Plants were grown in a greenhouse at 22 °C (day) and 18 °C (night); long-day photoperiods (16 h light/8 h darkness) were maintained with supplementary lighting (400 W Phillips HDK/400 HPI (R) (N). Plants were irrigated with a Hoagland No. 1 solution supplemented with oligoelements [39] . The origins of the veg1 / psfulc-1 , det-2, pim-1 and gigas-2 mutants have been previously described [11] , [16] , [17] , [40] . The psfulc-2 mutant was generated from line NGB5839 by EMS mutagenesis [27] . The psfulc-3 mutant was isolated by reverse screening in an EMS-mutagenized TILLING population of cultivar Caméor [28] . The veg2-1 mutant was isolated from fast-neutron mutagenesis of cv. Kaliski [41] . VIGS experiments [29] were performed on the cultivar Boneville. Each mutant was analysed in comparison with its corresponding parental wild-type line. Gene isolation and phylogenetic analysis The PsFULc complementary DNA was isolated from cDNA from inflorescence apices using PCR techniques; first, a 550-bp cDNA fragment was amplified by RT–PCR with primers derived from the M. truncatula FULc sequence and the remaining 5′- and 3′-fragments were amplified by PCR from a pea cDNA library [14] with primers from the vector and from the PsFULc cDNA fragment. To analyse the sequences of the PsFULc and PsSEP1 genes in the psfulc-2 mutant, several overlapping genomic fragments from each gene were amplified from genomic DNA from the mutant and from the parental wild type. All PCR fragments were cloned in pGEM-T easy (Promega) and sequenced. For the phylogenetic tree of the AP1/SQUA/FUL genes, the deduced amino acid sequences were aligned using the CLUSTALW tool in MACVECTOR 12.0 software (MacVector http://www.macvector.com/ ) and further refined by hand. Pairwise Poisson genetic distances were estimated from the alignment and a neighbour joining best tree was estimated using systematic tie-breaking and rooted to AMtrAGL2, an Amborella trichopoda orthologue of SEPALLATA. Mapping of PsFULc and PsSEP1 A population of 92 F 2 individuals from a cross between NGB5839 and JI1794 (Sussmilch et al ., unpublished) was used to map PsFULc and PsSEP1 in relation to other markers on the bottom of pea linkage group V. The description of the markers used is given in Supplementary Table S1 . No recombination was found between PsFULc and PsSEP1 , placing them 20 cM below COLa and 40 cM above FTb1 suggesting that they are less than 1 cM apart. TILLING To identify TILLING mutants in PsFULc , an EMS mutant population of 4,800 M2 families from Pisum sativum cultivar Cameor was screened. DNA isolation and pooling, PCR amplification and mutation detection were performed, as previously described [28] . For primer sequences in this and following sections in Methods see Supplementary Table S1 . PsFULc VIGS Two PsFULc -VIGS plasmids, pCAPE2-PsFULc193 and pCAPE2-PsFULc416, were used for the VIGS experiments. The pCAPE2-PsFULc193 and pCAPE2-PsFULc416 constructs derived from two non-overlapping PsFULc cDNA fragments of 193 bp (positions 166–359 from ATG) and 416 bp (positions 490–906 from ATG), respectively, which were generated by PCR and separately cloned into the VIGS vector pCAPE2, using Xba I and Bgl II cloning sites present in the PCR primers. The plasmid pCAPE2-Con, containing 400 bp of the GUS gene, was included for comparison as the VIGS control [42] . Inoculation of plants was carried out as previously described [29] with the following modifications. In each experiment, 12 plants were inoculated which each plasmid. At day 5 after inoculation, plants were decapitated and, for each plant, a single, basal, axial shoot was allowed to proliferate into a new primary shoot. At day 50 after decapitation, the newly outgrown primary shoot of each plant was analysed by scoring the number and nodal position of secondary inflorescences and of vegetative axial shoots exceeding 1 cm in length. Similar results were obtained in different experiments with each of the two PsFULc -VIGS plasmids; the data presented in the text corresponds to a representative experiment with the pCAPE2-PsFULc416 plasmid. Genotyping To discriminate between the wild-type and fulc-3 mutant alleles in the TILLING M3 family, we used a dCAPS marker with the primers FULc-dCF and FULc-dCR, which amplify a 228 bp fragment from the PsFULc gene (positions 2304–2532 from ATG at the PsFULc gene). FULc-dCF creates one mismatch generating a Sau3AI target site in the wild-type product (but not in psfulc-3 ), which after digestion produces two fragments of 26 bp and 202 bp. The veg1-1 single mutants and veg1-1 det-2 double mutants used for qPCR analysis were identified from segregating families. veg1-1 mutants were identified by absence of PCR product from primers FULc-2F and FULc-2R, which amplify a 950-bp fragment from the PsFULc gene, with primers TFL1a-1F and TFL1a-Rev03 used for a positive control PCR. det-2 mutants were determined using a CAPS marker with TFL1a-1F and TFL1a-Rev03 primers, which amplify a 764-bp fragment of the PsTFL1a/DET gene, which after digestion with EarI produces two fragments of 143 and 621 bp in the det-2 mutant because of the det-2 CAA-CGA substitution [15] . Southern analysis 10 μg of genomic DNA were digested with restriction enzymes and separated on 0.6%. TAE 1× agarose gels run overnight at 1 V cm −1 . Southern Blot analysis was performed by standard methods. The probe was a 550-bp fragment, amplified by PCR from the PsFULc cDNA (nucleotides 221–771 from the ATG) and cloned into the pGEM-T easy vector (Promega). RT–qPCR Total RNA was extracted using the SV Total RNA isolation system (Promega). RNA concentrations were determined by spectrophotometer analysis using a NanoDrop 8000 (Thermo Scientific). Reverse transcription was conducted in 20 μl with 1 μg of total RNA using the MMLV high-performance reverse transcriptase (Epicenter), according to the manufacturer's instructions. RT-negative (no enzyme) controls were performed to monitor for contamination with genomic DNA. First-strand cDNA was diluted 5 times, and 2 μl was used in each real-time PCR reaction. Real-time PCR reactions using SYBR green chemistry (Sensimix, Quantace, Bioline) were set up with a CAS-1200N robotic liquid handling system (Corbett Research) and run for 50 cycles in a Rotor-Gene RG3000 (Corbett). Two technical replicates and two-to-three biological replicates were performed for each sample. Relative transcript levels were evaluated using the reference gene ACTIN , as previously described [43] . In situ hybridization RNA in situ hybridization with digoxigenin-labelled probes was performed as described [44] . For PSFULc/VEG1 and DET , RNA antisense probes were generated using as substrate a 450-bp fragment of the PsFULc cDNA (236–686 from ATG) or a 460-bp fragment of the DET cDNA (358–818 from ATG), amplified by PCR and cloned into the pGEM-T Easy vector (Promega). For PIM , the probe was generated from a 767-bp of the 3′-region of the PIM cDNA, cloned into pGEM3Zf (Promega), as described [14] . Scanning electron microscopy (SEM) Samples for SEM were prepared and analysed as previously described [45] . Accession codes: The sequence data have been deposited in the NCBI GenBank database under accession codes JN974184 (PsFULC/VEG1 cDNA sequence) and JN974185 (PsFULC/VEG1 genomic sequence). How to cite this article: Berbel, A. et al . VEGETATIVE1 is essential for development of the compound inflorescence in pea. Nat. Commun. 3:797 doi: 10.1038/ncomms1801 (2012).